Female chromosome X mosaicism is age-related and preferentially affects the inactivated X chromosome To investigate large structural clonal mosaicism of chromosome X, we analysed the SNP microarray intensity data of 38,303 women from cancer genome-wide association studies (20,878 cases and 17,425 controls) and detected 124 mosaic X events >2 Mb in 97 (0.25%) women. Here we show rates for X-chromosome mosaicism are four times higher than mean autosomal rates; X mosaic events more often include the entire chromosome and participants with X events more likely harbour autosomal mosaic events. X mosaicism frequency increases with age (0.11% in 50-year olds; 0.45% in 75-year olds), as reported for Y and autosomes. Methylation array analyses of 33 women with X mosaicism indicate events preferentially involve the inactive X chromosome. Our results provide further evidence that the sex chromosomes undergo mosaic events more frequently than autosomes, which could have implications for understanding the underlying mechanisms of mosaic events and their possible contribution to risk for chronic diseases. Genetic mosaicism is classically defined as the coexistence of clonal cellular populations harbouring two or more distinct genotypes [1] . To date, detectable mosaicism has been reported in apparently healthy individuals as well as in patients with rare diseases, such as neurofibromatosis type II (NF2), trisomy 21, naevus sebaceous and Proteus syndrome [2] , [3] , [4] , [5] , [6] , [7] , [8] , [9] . Emerging data from consortia of genome-wide association studies (GWAS) [3] , [5] , [6] , [10] , [11] , [12] have demonstrated large autosomal mosaicism (events >2 Mb in size) in DNA collected from peripheral leukocytes and buccal epithelium. These studies suggest that autosomal mosaicism is associated with aging, hematologic cancer risk, and possibly ancestry and male sex. Whereas autosomal mosaicism is detectable in <2% of older individuals, recent studies indicate that large mosaic events may be far more common for the Y chromosome, and in particular among older men who smoke cigarettes [13] , [14] , [15] . The functional consequences of detectable chromosomal mosaicism remain to be fully determined. A number of groups have reported detectable genetic mosaicism of single-nucleotide mutations in the general population, particularly in genes implicated in hematopoietic disorders such as leukaemias and lymphomas [2] , [4] , [16] . Point-mutation events could reflect early, preleukemic clones and separately could increase risk for cardiovascular events [4] . Moreover, many reports have shown phenotypic consequences of chromosomal mosaicism that vary by genomic location of the event, developmental timing, tissue type involved and percentage of cells affected [7] , [8] , [9] . In prospective cohort studies, it has been possible to detect large mosaic structural events in blood samples of individuals who eventually develop chronic leukaemia, as early as 14 years before diagnosis, suggesting detection of a subset of events that eventually become manifest as part of the molecular profile of leukaemia [3] , [5] , [17] . To date, reports have not systematically addressed the frequency and characteristics of X chromosomal mosaicism. The X chromosome is unique among the human chromosomes in that normal women carry two copies and normal men carry one. To compensate for dosage differences between sexes, one copy of the female X chromosome is rendered transcriptionally inactive in a process called X inactivation [18] . In humans, the inactive X-chromosome (Xi) is randomly chosen early in development. Once established, X inactivation is generally irreversible and stably maintained through mitotic divisions. Established mechanisms for maintaining X inactivation include expression of the non-coding XIST RNA, chromatin modifications, changes in nuclear scaffold proteins, and DNA methylation [19] , [20] , [21] , [22] , [23] . Sequence data from cancer genomes suggest that the X chromosome, particularly the female Xi, has a higher somatic mutation load of point mutations than the autosomes [24] . It has been postulated that the observed higher load of somatic point mutations could be directly related to the timing of Xi replication, which occurs late and is faster than either the active X-chromosome (Xa) or the autosomes [25] , [26] , [27] . Although these and other data suggest that X-chromosome mosaicism may be detectable at a prevalence higher than that observed on the autosomes [28] , [29] , [30] , little is known about its frequency in the population or basic characteristics of the distribution and types of gains, losses and acquired loss of heterozygosity. In this report, we investigate the frequency of large-scale chromosome X mosaicism (>2 Mb) in blood or buccal samples from 38,303 women. We observe an overall frequency of X mosaicism of ∼ 0.25%, roughly four times the mean autosomal rate. The frequency of X mosaicism increases with increasing age, but is not associated with non-haematologic cancer risk. Further investigations by methylation analyses suggest the inactive X chromosome is preferentially gained or lost in X mosaic events. Detected chromosome X events Using a segmentation algorithm, we conducted a systematic scan of large structural detectable mosaicism on the X chromosomes of 38,303 women (20,878 cancer cases and 17,425 cancer-free controls), who had been previously examined for autosomal mosaicism [3] , [11] , [12] . 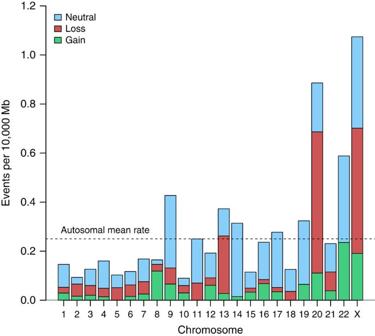Figure 1: Adjusted mean rate of events by chromosome. A comparison of detected mosaic events >2 Mb in size in the autosomes to the X chromosome (X events=124, Autosomal events=430). 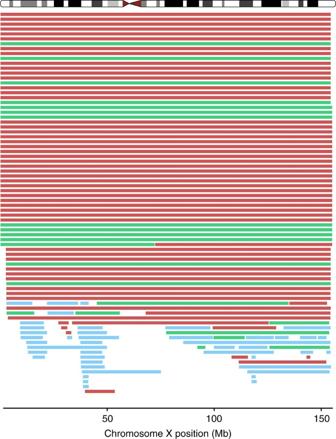Figure 2: Detected mosaic events on the X chromosome. Mosaic losses (N=59) are in red, mosaic gains (N=22) are green, and mosaic copy-neutral events (N=43) are in blue. In total, 124 mosaic events greater than 2 Mb in size were detected on the X chromosomes of 97 of the 38,303 women who were scanned (0.25%, Supplementary Table 1 , Supplementary Table 2 ); all detected cases of trisomy X and XO (Turner’s syndrome) were removed from subsequent analyses ( n =5). Of the 97 women with detected X events, 15 (15%) had more than one event detected on their X chromosome, with one woman having as many as five events. The base-pair adjusted rate of mosaic X events was 1.07 events per 10,000 Mb, over fourfold higher than the mean 0.25 events per 10,000 Mb rate observed across the autosomes [12] ( P value=1.32 × 10 −5 , Fig. 1 ). Significantly elevated rates were observed for the X chromosome in comparison with all autosomes except for chromosome 20 (chr20=0.89, chrX=1.07 events per 10,000 MB; P value=0.29). The 124 mosaic X events consisted of 59 mosaic losses, 43 mosaic copy-neutral events and 22 mosaic gains ( Fig. 2 , Supplementary Fig. 1 ). These events mostly included the whole chromosome, with a fraction (37%) mapping to the interstitial region ( Table 1 ). Few events were found at either the centromeric or telomeric ends. Most whole-X-chromosome events were mosaic losses. 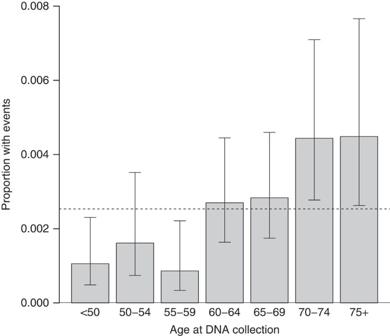Figure 3: Unadjusted age relationship with X mosaicism. Dashed line represents the mean overall proportion with mosaic X events across all age groups and error pars represent 95% Wilson confidence intervals (N=31,982). Interstitial events were primarily mosaic copy-neutral loss of heterozygosity, which have been less extensively documented in the cytogenetic literature on chromosome X ( Supplementary Table 3 ). Two notable clusters of interstitial mosaic copy-neutral events are centered at approximately 26 and 49 Mb (NCBI36/hg18, Fig. 2 ). While X-chromosome mosaic events were more common than autosomal events, the mean proportion of cells with X-chromosome mosaicism tended to be lower than the mosaic proportion with autosomal events overall (X=0.299, autosomes=0. 359, P value=0.01, Supplementary Fig. 2 ), however, this association was not observed in cancer-free individuals ( P value=0.10). Women with an X-chromosome mosaic event had a significantly higher likelihood of harbouring an autosomal event relative to women without detectable X mosaicism (unadjusted odds ratio (OR unadj )=16.7, 95% confidence interval (CI)=8.3-33.6, P value=2.5 × 10 −15 ), even after adjusting for age (adjusted odds ratio (OR adj )=15.6, 95% CI=7.3-33.0, P value=8.6 × 10 −13 ). Figure 1: Adjusted mean rate of events by chromosome. A comparison of detected mosaic events >2 Mb in size in the autosomes to the X chromosome (X events=124, Autosomal events=430). Full size image Figure 2: Detected mosaic events on the X chromosome. Mosaic losses ( N =59) are in red, mosaic gains ( N =22) are green, and mosaic copy-neutral events ( N =43) are in blue. Full size image Table 1 Chromosomal arm location of detected mosaic autosomal and X events. Full size table Validation by qPCR Detected X mosaic events were experimentally validated using a set of 12 quantitative PCR assays (qPCR) across chromosome X. Specifically, we estimated copy-number ratios for 26 events across 25 females with single-nucleotide polymorphism (SNP) microarray-detected X mosaicism with a range of mosaic proportions from 6 to 88%. In the 18 mosaic samples with events that spanned the entire X chromosome, the concordance rate was 100% for gains and 80% for losses ( Supplementary Table 5 ). An inspection of the discordant copy-loss samples called as copy-neutral events revealed qPCR copy-number values near the calling threshold, or samples with low mosaic proportions. For detected mosaic events spanning only a portion of the X chromosome, four of the eight (50%) showed evidence for mosaic copy-number changes by qPCR, although only 25% were concordant in copy-number state with qPCR ( Supplementary Table 5 ), suggesting the limited subsets of qPCR probes that spanned events may have been insufficient to adequately call copy-number states. X mosaicism in men We also examined X-chromosome mosaicism in men. Although we identified 187 men with suggestive evidence of X-chromosome mosaicism (from 43,735 scanned participants), results from qPCR validation in 39 men with available DNA were poor (15% concordance). Calling X-chromosome mosaicism is inherently more challenging in men as their possession of a single X-chromosome precludes analysis with the B-allele frequency (BAF). Although certainly of interest, further refinement of the calling algorithm is required before we can reliably call detectable X mosaicism in men. All subsequent analyses of X mosaicism reported herein are restricted to women. X mosaicism associations Detectable X mosaicism increases with age, with more events in older women than in younger women. The estimated frequency of X mosaicism was 0.11% in women under 50 years of age and 0.45% in women 75 years or older ( Fig. 3 ). Multivariate analyses adjusted for ancestry, cancer status and study found a statistically significant association with an OR of 1.04 per 1-year increase in age (95% CI=1.01–1.06, P value=0.005), with a 20-year increase in age resulting in over twice the odds of a acquiring a mosaic event on the X chromosome. Altogether with prior evidence from autosomes and the Y chromosome [12] , [13] , our data suggest that each human chromosome is susceptible to age-related structural deterioration related to clonal mosaicism, but at distinct rates. Y mosaic events are more common than X events, and X events are more common than those in autosomes. These frequencies may reflect intrinsic differences in the mechanisms by which each type of chromosome is replicated or protected against age-related DNA damage [26] . Figure 3: Unadjusted age relationship with X mosaicism. Dashed line represents the mean overall proportion with mosaic X events across all age groups and error pars represent 95% Wilson confidence intervals ( N =31,982). Full size image Comparable to what we reported for the autosomes (in over 127,000 individuals scanned), we found little to no evidence for an overall association between X mosaicism and non-haematologic cancer ( P value=0.19) [3] , [5] , [12] . An analysis by cancer site found at most a marginally significant association between X mosaicism and lung cancer risk (OR=1.89, 95% CI=1.02–3.50, P value=0.042; 26 lung cancer cases with mosaicism). However, we had only a limited sample size, were unable to adequately adjust for the major lung cancer risk factor, cigarette smoking and we did not consider multiple comparisons across cancer types. We did not detect an association between X mosaicism and ancestry (three continental populations: European, African and East Asian, P value=0.40) that was detected in prior autosomal mosaicism analyses [12] . In addition, we did not find evidence for an association between X mosaicism and smoking for a subset of women with available smoking information ( N =19,197, ever smoker versus never smoker P value=0.54). Interestingly, an association was found between DNA source and X mosaicism in which X mosaicism was more frequent in buccal cells as compared with leukocytes (OR=3.50, 95% CI=1.45–8.46, P value=0.005). Larger studies are required to confirm these findings. Methylation analysis To investigate the molecular basis of X-chromosome mosaicism, we used Illumina HumanMethylation450 microarray data for a subset of mosaic females with sufficient DNA to determine whether mosaic events are preferential for either the Xa or Xi. Established sex-specific differences in chromosome X promoter methylation [31] , [32] provide an opportunity to determine whether the pattern of large structural mosaic events parallels what has previously been reported for analyses of somatic mutations in cancer, namely, events more likely occurring in the inactive X-chromosome [24] . After we completed a rigorous quality control process for methylation microarray data in a control population of 1,665 men and 136 women, probes in gene promoter sites on the X chromosome were extracted and filtered to focus analyses on a reference set of probes that were differentially methylated between men and women, as these are the locations that are inactivated on Xi ( Supplementary Fig. 3 ) [31] , [32] . Methylation beta values for the resulting set of 1,888 probes were evaluated for differences from normal expected values in women (beta values greater than expected suggest mosaic gain of Xi and less than expected suggest mosaic loss of Xi) ( Fig. 4 ). Of the 21 women with mosaic losses, 16 had evidence for a loss of the Xi chromosome. Similarly, all 5 women with mosaic gains had evidence suggesting a mosaic gain of Xi. For mosaic copy-neutral events, 6 women showed evidence for a loss of a portion of the Xa and a replacement with Xi and one woman showed evidence for a loss of a portion of Xi and a replacement with the Xa. Our combined data for mosaic gains and losses suggest that Xi is preferentially involved in mosaic copy-number changes, with Xi more commonly altered in mosaic losses and preferentially gained for mosaic gains ( P value=0.002). Mosaic events on the X chromosome that do not follow this trend, particularly the five mosaic losses with evidence for a loss of the Xa, could represent normal variation, perhaps due to different DNA extraction techniques, noise in the methylation assay or statistical outliers. Alternatively, chromosome X events could occur early in female development, perhaps at a time that precedes X-inactivation, and thus X-inactivation could only occur in cells with more than one X chromosome. 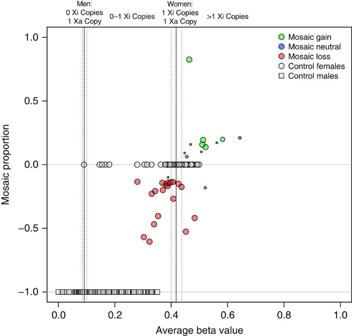Figure 4: Chromosome X methylation beta values by estimated mosaic proportion. Average beta values (range: 0.0–1.0) indicate amount of methylation at a genomic locus where low values indicate hypomethylation and high values indicate hypermethylation. X methylation beta values are plotted for promoter probes spanning a mosaic X event and points are sized for the number of probes. The estimated mosaic proportion is calculated from the mosaic proportion estimate of the SNP microarrays and direction (positive versus negative) is determined from average probe betaz-scores. Control men (N=1,665) and women (N=136) are shown as light grey squares and circles. Mosaic females (N=48) are plotted as green, blue and red circles for mosaic gains, copy-neutral events and losses, respectively. Solid and dashed black lines are median and interquartile range for control men (left) and women (right) beta values. Figure 4: Chromosome X methylation beta values by estimated mosaic proportion. Average beta values (range: 0.0–1.0) indicate amount of methylation at a genomic locus where low values indicate hypomethylation and high values indicate hypermethylation. X methylation beta values are plotted for promoter probes spanning a mosaic X event and points are sized for the number of probes. The estimated mosaic proportion is calculated from the mosaic proportion estimate of the SNP microarrays and direction (positive versus negative) is determined from average probe beta z -scores. Control men ( N =1,665) and women ( N =136) are shown as light grey squares and circles. Mosaic females ( N =48) are plotted as green, blue and red circles for mosaic gains, copy-neutral events and losses, respectively. Solid and dashed black lines are median and interquartile range for control men (left) and women (right) beta values. Full size image Our analysis using SNP microarray intensities identified detectable mosaic events on the female X chromosome that occur at higher frequencies than mosaic events on the autosomes. We observed evidence that individual women with mosaic events of the X chromosome are also more likely to have mosaic events of the autosomes. Furthermore, X mosaic events are more likely to involve the inactive X chromosome than the active X chromosome, and thus might be phenotypically neutral. As with autosomal and Y mosaicism, X mosaicism increases with age. For decades, it has been apparent that an appreciable fraction of paediatric developmental disorders are directly attributable to a spectrum of mosaic events (for example, from point mutations to large structural alterations) that can also influence clinical course [9] , [33] , [34] , [35] . Our data indicate that substantial numbers of adults also possess mosaic chromosomes in blood and buccal cells, suggesting the genome undergoes somatic alterations that either are generated later due to less efficient protective mechanisms or were perhaps tolerated from early age and subsequently expanded due to less efficient mechanisms for retaining genomic stability. A limitation of our analysis is the low level of validation for partial chromosome copy-neutral events. Because of both the smaller event size and the need for log R ratio (LRR) baseline correction, our array-based detection algorithm together with qPCR-based validation yielded a low level of concordance. Further work is needed to improve the calling algorithms, which could also be accelerated by the analysis of larger samples sizes, ultimately leading to more precise measurement of mosaic X-chromosomal events. It is striking that the frequency of large megabase mosaicism is higher in the inactive X as well as the Y chromosome compared with the autosomes. This higher frequency of mosaicism on sex chromosomes could be a reflection of less cell selection because the inactive X is transcriptionally inactive while the Y chromosome has the smallest number of genes. Future studies are needed to understand the mechanisms responsible for the generation and selection of these mosaic alterations in sex and autosomal chromosomes, which occur at different frequencies. In turn, insights into the underlying mechanisms as well as the differences in frequencies of large structural genetic mosaicism should provide an important foundation for understanding their contribution to health and chronic diseases [6] , [36] , [37] . Study population The data set was drawn from cancer GWAS of solid tumours performed at the National Cancer Institute Division of Cancer Epidemiology and Genetics and the Cancer Genome Research Laboratory. In total, peripheral leukocyte or buccal epithelial DNA was available for 20,878 solid tumour cancer cases and 17,425 cancer-free controls. DNA was genotyped on one or more commercially available Illumina Infinium Human SNP array (Hap300, Hap240, Hap550, Hap610, Hap660, Hap 1, Omni Express, Omni 1, Omni 2.5 and Omni 5). Quality control procedures were applied after genotyping and samples were clustered in batches to optimize accuracy and minimize batch effects. All GWAS studies were reviewed by the Institutional Review Board of the National Cancer Institute and those of the participating study centers. Informed consent was received for each study participant before study enrollment. Detection algorithm BAF and LRR are two metrics used to detect mosaic events. BAF is a measure of allelic imbalance and used to quantify deviation of an individual’s SNP genotype from expected AA, AB and BB genotype clusters. Contiguous runs of heterozygous SNPs with BAF values that deviate from the expected value of 0.5 are evidence for mosaicism. The LRR value of an individual’s SNP is a proxy for copy number. LRR values are the log 2 of the ratio of observed SNP intensity value to expected intensity value. LRR values greater than expected baseline LRR suggest copy gain and less than expected baseline LRR suggest copy loss. The expected baseline LRR was calculated from women within each clustering group based on the ratio of males and females in the original genotyping cluster group. All BAF and LRR values were calculated using methods described [38] and renormalized as outlined previously [3] . For female participants, BAF and LRR values were systematically scanned across the X chromosome. Chromosomes were segmented for mosaic events using circular binary segmentation (CBS) on BAF values with the BAF segmentation package [39] . Segments <2 Mb in size were filtered out to control the false-positive rate. Gaussian mixture models were fit to BAF bands to assign event type given the best-fitting model (2–4 Gaussian components). Event copy-number state was assigned based on LRR values with baselines adjusted for the number of men present within original genotyping cluster groups. For whole-chromosome mosaic X events, LRR deviations of 0.01 and −0.01 were used to classify events as gain and losses, respectively. For mosaic X events encompassing only a portion of the X chromosome, we chose a more conservative threshold of 0.05 and −0.05 for gains and losses due to greater LRR variation due to the reduced number of X probes that spanned the events. Mosaic proportions were estimated using deviation from the expected BAF given the LRR defined copy-number state. Further details are outlined in our prior work on autosomal mosaicism [3] . Quantitative PCR qPCR assays were selected to determine copy-number status of 12 regions spanning the X chromosome by normalizing to an autosomal gene, RNase P, which is present in two copies in a diploid genome ( Supplementary Table 4 ). One additional assay was run to validate the presence of the Y chromosome. According to Quant-iT PicoGreen dsDNA quantitation (Life Technologies, Grand Island, NY), 5 ng of sample DNA were transferred into LightCycler-compatible 384-well plates (Roche, Indianapolis, IN) in triplicate and dried down. Two internal standard curves were run separately in each plate, pooled gDNA samples of males and pooled gDNA samples of females, both with no detectable X chromosome loss/gain, and serially diluted to 6 concentrations. qPCR was performed using 5 μl reaction volumes consisting of: 2.5 μl of LightCycler 480 Probes Master Mix (Roche, Indianapolis, IN), 2.0 ul of MBG Water, 0.25 μl of 20 × TaqMan Copy Number Reference Assay, RNase P (Life Technologies, Grand Island, NY), and 0.25 μl of specific 20 × TaqMan Copy Number Assay (Life Technologies, Grand Island, NY). Thermal cycling was performed on a LightCycler 480 (Roche) where PCR conditions consisted of: 95 °C hold for 5 min, denature at 95 °C for 15 s, anneal at 60 °C for 30 s, with fluorescence data collection over 45 cycles. All experimental and control samples were assayed in triplicate on each plate, separately for all 12 individual target assays. The LightCycler software (Release 1.5.0) was used for initial analysis of the raw data, utilizing the absolute quantification analysis with the second derivative maximum method and high-confidence detection algorithm, to yield a crossing threshold (Ct) for all replicates. The Ct for each assay was used to interpolate concentration of target and reference sequences using the standard curves. The ratio of target to reference was multiplied by 2 to determine the diploid amount of X chromosome in that region. The ratios of the 12 assays were then averaged to yield an overall X-chromosome signal ratio. Seventy-five normal copy-number controls were used to estimate normal probe ratio means and s.d. A value of 3 s.d. above the normal mean ratio was used as the threshold to call gains and a value of 3 s.d. below the normal mean ratio was the threshold for calling losses. Methylation arrays After Quant-iT PicoGreen dsDNA quantitation (Life Technologies, Grand Island, NY), 1,000 ng of sample DNA were treated with sodium bisulfite using the EZ-96 DNA Methylation MagPrep Kit (Zymo Research, Irvine, CA) to convert unmethylated cytosine residues to uracils (detected as thymidines), leaving 5′-methylcytosines residues unaffected. Bisulfite-treated samples were denatured, neutralized and then whole-genome amplified, isothermally, to increase the amount of DNA template. The amplified product was enzymatically fragmented, precipitated and resuspended in hybridization buffer. Samples were hybridized overnight on Infinium HumanMethylation450 BeadChips (Illumina Inc., San Diego, CA), which allowed fragmented DNA to anneal to locus-specific 50mers (covalently linked to one of over 500,000 bead types). Single-base extension of oligonucleotides on the BeadChip, using the captured DNA as template, incorporated tagged nucleotides on the BeadChip, which were subsequently fluorophore labelled during staining. BeadChips were scanned by an Illumina iScan at two wavelengths to create image and intensity files. An internal control, a DNA sample from a lymphoblastoid cell line NA07057 (Coriell Cell Repositories, Camden, NJ), was utilized to confirm the efficiency of bisulfite conversion and subsequent methylation analysis. Methylation beta values are indicators of site-specific methylation with a theoretical range from 0 to 1, where low values indicate hypomethylation and high values indicate hypermethylation. Raw beta intensity values were extracted for probes in promoter sites on the X chromosome and further filtered to include only probes that are differentially methylated between women (Xa/Xi) and men (Xa). A control sample of available men ( N =1,665) and women ( N =136) was used to determine expected beta value means and s.d. Using the RnBeads R library, promoter probes were selected that had mean beta values between 0.35 and 0.5 and s.d. <0.09 in women and mean beta values <0.15 and s.d. <0.05 in men ( Supplementary Fig. 3 ). This left a total of 1,888 differentially methylated probes that spanned 212 promoter sites across the X chromosome for analysis. For each mosaic female, mean beta values and z-scores were calculated for all differentially methylated promoter probes that spanned detected mosaic X events in an effort to determine changes in methylation profiles and thus phase mosaic events to the Xa or Xi chromosomes. The mosaic proportions were calculated from SNP microarray per cent mosaicism values. Only X events spanning 5 or more promoter regions were used for the analysis. Statistical analysis All statistical analyses were performed on a 64 bit Windows build of R 3.0.1 "Good Sport". Multivariate analyses used logistic regression models (glm procedure) with X mosaicism as the dependent variable and adjusted for age of DNA collection, study indicator variables, cancer status (case=1, control=0), and genetically inferred ancestry (%European, %African and %Asian) unless otherwise specified. Inferred ancestry proportions were estimated for each individual using reference populations from the HapMap project [40] with the GLU software package ( https://code.google.com/p/glu-genetics/ ) using the struct.admix module. Confidence intervals for plots are Wilson intervals. All reported P values are two-sided. Data availability Original study data has been posted in dbGaP ( http://www.ncbi.nlm.nih.gov/gap ) under accession numbers phs000093.v2.p2, phs000336.v1.p1, phs000351.v1.p1, phs000361.v1.p1, phs000652.v1.p1, phs000716.v1.p1, phs000734.v1.p1, phs000396.v1.p1, phs000147.v2.p1, phs000346.v2.p1, phs000863.v1.p1 and phs000206.v5.p3. Data on called event features, location and individual characteristics are available in Supplementary Table 1 . Methylation array beta values for events are presented in Supplementary Table 6 and raw data is posted in dbGaP under accession number phs001112.v1.p1. The methylation data has been deposited in dbGaP under accession code phs001112.v1.p1 How to cite this article: Machiela, M.J. et al . Female chromosome X mosaicism is age-related and preferentially affects the inactivated X chromosome. Nat. Commun. 7:11843 doi: 10.1038/ncomms11843 (2016).